Carrier localization and electronic phase separation in a doped spin-orbit-driven Mott phase in Sr3(Ir1–xRux)2O7 Interest in many strongly spin-orbit-coupled 5d -transition metal oxide insulators stems from mapping their electronic structures to a J eff =1/2 Mott phase. One of the hopes is to establish their Mott parent states and explore these systems’ potential of realizing novel electronic states upon carrier doping. However, once doped, little is understood regarding the role of their reduced Coulomb interaction U relative to their strongly correlated 3 d -electron cousins. Here we show that, upon hole-doping a candidate J eff =1/2 Mott insulator, carriers remain localized within a nanoscale phase-separated ground state. A percolative metal–insulator transition occurs with interplay between localized and itinerant regions, stabilizing an antiferromagnetic metallic phase beyond the critical region. Our results demonstrate a surprising parallel between doped 5 d - and 3 d -electron Mott systems and suggest either through the near-degeneracy of nearby electronic phases or direct carrier localization that U is essential to the carrier response of this doped spin-orbit Mott insulator. Iridium 4+ ions with a half-filled 5 d shell in a cubic octahedral oxygen coordination occupy a unique region in relative energy scales: one where a model of crystal field splitting combined with strong spin-orbit coupling (SOC) breaks the fivefold degeneracy of electronic states into fully occupied J eff =3/2 and half-filled J eff =1/2 bands [1] , [2] . The resulting bandwidth-narrowed J eff =1/2 states allow the relatively modest U (~1.5–2 eV) inherent to these 5 d -transition metal elements [3] to split the band and generate a charge gap. A SOC-assisted Mott phase results, allowing an unexpected manifestation of correlation-driven physics in materials with extended 5 d -electron wave functions. Doping this spin-orbit Mott phase has since generated predictions of stabilizing states analogous to those found in doped strongly correlated 3 d -electron Mott insulators such as the high-temperature cuprate superconductors [4] . To date however, the role of Coulomb interactions in the doped J eff =1/2 Mott phase remains contentious with no direct observations of correlated electronic phase behaviour. Two prototypical spin-orbit Mott materials are the n =1 and n =2 members of the iridate Ruddelsden–Popper series Sr n +1 Ir n O 3 n +1 (refs 5 , 6 ). Here the bilayer system Sr 3 Ir 2 O 7 (Sr-327) possesses a low-temperature charge gap of E g =130 meV, [7] roughly reduced by a factor of four from the gap of its single-layer cousin Sr 2 IrO 4 (ref. 8 ). This reduced gap renders the Sr-327 system a fortuitous starting point for perturbing the spin-orbit Mott phase and exploring carrier-induced electronic phase behaviour as the system is driven toward the metallic regime. To this end, in this work Ru 4+ (4 d 4 ) ions are substituted onto the Ir 4+ (5 d 5 ) sites of Sr 3 (Ir 1− x Ru x ) 2 O 7 with the known end point, Sr 3 Ru 2 O 7 , possessing a Fermi liquid ground state in close proximity to a magnetic instability [9] . Our combined transport, magnetization, neutron scattering and scanning-tunnelling spectroscopy (STS) studies show that the Mott insulating state of Sr 3 Ir 2 O 7 is remarkably robust as the in-plane doped holes remain largely localized within a nanoscale phase-separated ground state and only generate a metal–insulator transition (MIT) near the two-dimensional (2D) percolation threshold. The resulting electronic phase diagram also reveals the surprising persistence of antiferromagnetic (AF) order deep into the metallic phase and suggests emergent itinerant magnetism at the interface between the AF-ordered spin-orbit Mott phase of Sr 3 Ir 2 O 7 and the nearly magnetic Fermi liquid electronic phase of Sr 3 Ru 2 O 7 . Electronic phase diagram and bulk electronic properties The resulting electronic phase diagram determined via our combined transport, bulk magnetization and neutron-scattering measurements is plotted in Fig. 1a . The most prominent feature of the phase diagram is that the transition from the insulating ground state of Sr 3 Ir 2 O 7 to the low-temperature metallic phase takes place only beyond the critical concentration of x =0.35. This suggests that the Ir 4+ (5 d 5 ) valence is protected by the Mott gap that blocks the charge transfer of doped holes from the in-plane substituted Ru 4+ (4 d 4 ) ions, a phenomenon of ‘Mott blocking’. The corresponding resistivity ρ ( T ) is plotted as a function of temperature in Fig. 2a for Sr 3 (Ir 1− x Ru x ) 2 O 7 concentrations spanning the phase diagram. Concentrations near the phase boundary also show a thermally driven MIT as illustrated in the inset of Fig. 2a for x =0.33 with T MIT =135 K (see also Supplementary Fig. 1 ). As an initial window into the corresponding evolution of the magnetic order, the high-temperature inflection in ρ ( T ) in the x =0 parent compound is known to identify the onset of canted AF order at T AF =280 K. This feature in ρ ( T ) is gradually suppressed to lower temperatures upon Ru doping, where the anomaly vanishes in the metallic regime. 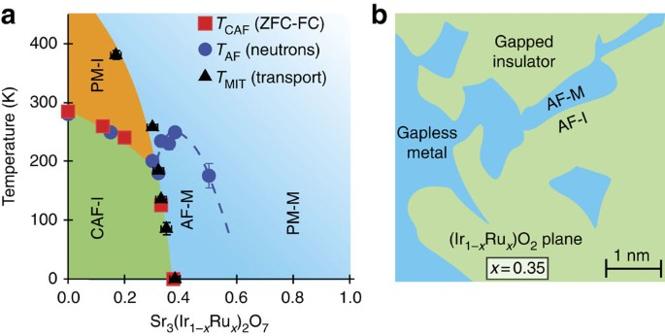Figure 1: Electronic phase diagram of Sr3(Ir1−xRux)2O7. (a) Evolution of electronic phases of Sr3(Ir1−xRux)2O7as a function of Ru concentration. CAF-I denotes the insulating canted AF phase, PM-I denotes the paramagnetic insulating phase, AF-M denotes the AF ordered metallic state and PM-M indicates the paramagnetic metallic regime. Squares indicate the onset of canted AF order determined with bulk susceptibility measurements, circles denote the onset of AF order as observed via neutron direction measurements, and triangles indicate the transition temperatures for thermally driven MITs near the phase boundary. (b) Illustration of the basal-plane showing phase-separated metallic puddles near the percolative threshold, which nucleate within the spin-orbit Mott insulating background of Sr3Ir2O7. Error bars in all plots represent 1 s.d. Figure 1: Electronic phase diagram of Sr 3 (Ir 1− x Ru x ) 2 O 7 . ( a ) Evolution of electronic phases of Sr 3 (Ir 1− x Ru x ) 2 O 7 as a function of Ru concentration. CAF-I denotes the insulating canted AF phase, PM-I denotes the paramagnetic insulating phase, AF-M denotes the AF ordered metallic state and PM-M indicates the paramagnetic metallic regime. Squares indicate the onset of canted AF order determined with bulk susceptibility measurements, circles denote the onset of AF order as observed via neutron direction measurements, and triangles indicate the transition temperatures for thermally driven MITs near the phase boundary. ( b ) Illustration of the basal-plane showing phase-separated metallic puddles near the percolative threshold, which nucleate within the spin-orbit Mott insulating background of Sr 3 Ir 2 O 7 . Error bars in all plots represent 1 s.d. 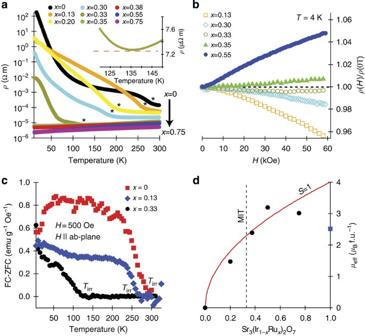Figure 2: Bulk transport and magnetization measurements of Sr3(Ir1−xRux)2O7. (a) Resistivity plotted as a function of temperature for Ru concentrations spanning the MIT. Inset shows thermally driven transition atTMIT=135 K forx=0.33. (b) 4 K magnetoresistance plotted as a function of applied field for Ru concentrations spanning the MIT. (c) Field-cooled (FC) minus zero-field cooled (ZFC) magnetization as a function of temperature for select Ru dopings. (d) Local moments extracted from Curie–Weiss fits plotted as a function of Ru concentration. Solid line denotes the expected full moment value forS=1 impurities. The blue square denotes data taken from Ikedaet al.111 emu g−1Oe−1=4π × 10−3m3kg−1. Error bars in all plots represent 1 s.d. Full size image Figure 2: Bulk transport and magnetization measurements of Sr 3 (Ir 1− x Ru x ) 2 O 7 . ( a ) Resistivity plotted as a function of temperature for Ru concentrations spanning the MIT. Inset shows thermally driven transition at T MIT =135 K for x =0.33. ( b ) 4 K magnetoresistance plotted as a function of applied field for Ru concentrations spanning the MIT. ( c ) Field-cooled (FC) minus zero-field cooled (ZFC) magnetization as a function of temperature for select Ru dopings. ( d ) Local moments extracted from Curie–Weiss fits plotted as a function of Ru concentration. Solid line denotes the expected full moment value for S =1 impurities. The blue square denotes data taken from Ikeda et al . [11] 1 emu g −1 Oe −1 =4π × 10 −3 m 3 kg −1 . Error bars in all plots represent 1 s.d. Full size image Low-temperature magnetoresistance (MR) data with the magnetic field applied perpendicular to the ab plane are plotted in Fig. 2b . The negative magnetoresistance previously reported in the parent material [10] and indicative of suppressed spin fluctuations or magnetic domain scattering persists in lightly doped, insulating samples; however, as the system transitions into the metallic phase, the MR smoothly switches sign from negative to positive values that increase in magnitude with continued Ru doping. This suggests that orbital (Lorentz force) effects begin to dominate across the MIT phase boundary as the carrier concentration is enhanced while fluctuation/domain effects from AF order are damped. Further illustrating this, bulk magnetization measurements of the in-plane susceptibility were performed on select samples, shown in Fig. 2c . As Ru is doped into Sr-327, the onset temperature of the net ferromagnetism, arising from the canted AF order and denoted via the irreversibility temperature ( T irr ), is reduced. Close to the critical regime, the x =0.33 sample exhibiting a thermally driven MIT with T MIT =135 K ( Fig. 2a inset) shows an onset of canted AF order at the same temperature. This suggests that near the MIT phase boundary the two transitions ( T MIT and T CAF ) become coupled and that this coupling diminishes in lightly doped samples deeper within the insulating regime. Samples with Ru doping x >0.33 show no irreversibility in magnetization, and concentrations with a metallic ground state show only local moment behaviour within resolution. The only exception is that the highest doped sample with x =0.75 shows the reemergence of T irr at low temperature ( Supplementary Fig. 2 ); however, the origin of this may simply be an extrinsic perturbation of the nearby Fermi liquid phase of Sr 3 Ru 2 O 7 . Through direct analogy with Sr 3 Ru 2 O 7 (ref. 11 ), Ru nominally enters the Sr-327 iridate lattice in the low spin state of Ru 4+ and subsequently introduces S =1 impurities into the J eff =1/2 magnetic background. Unlike its single-layer cousin Sr 2 IrO 4 (ref. 12 ), the parent Sr-327 iridate shows no Curie–Weiss behaviour up to 400 K [13] ; however, as Ru ions are introduced into the lattice a paramagnetic upturn begins to build in the low-temperature magnetization data for the lowest doping measured ( x =0.13). Immediately upon doping Ru, the known low-temperature downturn in χ( T ) in the parent system [10] , [14] ( Fig. 2c ) rapidly vanishes and is replaced by a weak paramagnetic upturn. The resulting local moments, extracted via Curie–Weiss fits to the susceptibility, are plotted in Fig. 2d . For low Ru-dopant levels, the effective local moments extracted from each concentration track the expectation for contributions solely arising from local S =1 impurities, which build continuously across the MIT. This suggests Ru ions remain largely localized at low Ru dopings within the insulating background of Sr 3 Ir 2 O 7 and that their survival into the metallic regime demonstrates robust correlation effects on either side of the MIT. For doping levels beyond x =0.5, the local moments are screened and smoothly connect to the high-temperature susceptibility of metallic Sr 3 Ru 2 O 7 (ref. 11 ). Neutron-scattering measurements In order to more directly elucidate the evolution of the ordered AF phase across the MIT in this system, neutron-scattering measurements were performed. The results plotted in Fig. 3a show that, for insulating samples, the onset of long-range AF order coincides with the T irr determined via the magnetization curves in Fig. 2 . Upon increased doping, however, the AF phase surprisingly survives across the MIT at the same Q positions as the insulating phase [10] , [15] , and the resulting order parameters for metallic samples are plotted in Fig. 3b . From the limited number of magnetic peaks observable in our neutron measurements ((1, 0, L ); L =1, 2, 3, 4), the spin structure remains consistent with that of the parent system across the MIT in the phase diagram, albeit the small degree of spin canting present in the insulating parent system is necessarily eliminated or strongly suppressed in the metallic regime. The persistent AF order remains long-range within resolution with a minimum correlation length ξ ≈200 Å ( , where w is obtained by fits of radial scans to the form ). Keeping a model of c axis-aligned moments across the MIT [5] , Fig. 3c , shows a nearly linear suppression of the AF moment in the lightly Ru-doped insulating regime due to the dilution of ordered Ir ions by localized Ru S =1 impurities, and deep in the metallic regime the ordered moment is quickly screened. In close proximity to the MIT phase boundary however, an anomalous enhancement in the ordered AF moment appears ( Fig. 3 and Supplementary Fig. 3 ), suggesting the potential of induced ordering of S =1 moments from doped 4 d 4 electrons in this range or potentially a partial relaxation of the octahedral distortion resulting in enhanced magnetic exchange. 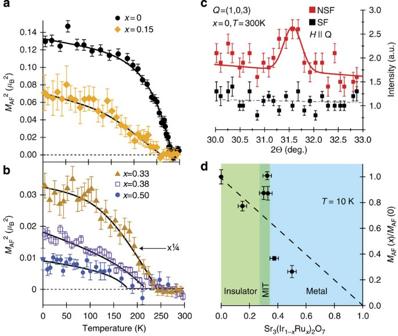Figure 3: Neutron scattering characterization of Sr3(Ir1−xRux)2O7. (a) Temperature evolution of the square of the AF order parameter (MAF2(T)) for fully insulatingx=0 (from ref.10) andx=0.15. (b)MAF2(T)for metallicx=0.5 andx=0.38 samples as well as forx=0.33 at the phase boundary. The data forx=0.33 have been scaled by ¼ for clarity. (c) Ordered AF moments for Sr3(Ir1−xRux)2O7scaled relative to the parent Sr3Ir2O7insulator. Shaded areas denote boundaries between insulating, metallic and critical MIT regimes. (d) Polarized neutron diffraction measurements of Sr3Ir2O7showing radial scans through theQ=(1, 0, 3) superlattice peak at 300 K in both spin-flip (SF) and non-spin-flip (NSF) channels. The magnetic guide field was applied parallel to the momentum transferQ. Error bars in all plots represent 1 s.d. Figure 3: Neutron scattering characterization of Sr 3 (Ir 1− x Ru x ) 2 O 7 . ( a ) Temperature evolution of the square of the AF order parameter ( M AF 2 ( T )) for fully insulating x =0 (from ref. 10 ) and x =0.15. ( b ) M AF 2 (T) for metallic x =0.5 and x =0.38 samples as well as for x =0.33 at the phase boundary. The data for x =0.33 have been scaled by ¼ for clarity. ( c ) Ordered AF moments for Sr 3 (Ir 1− x Ru x ) 2 O 7 scaled relative to the parent Sr 3 Ir 2 O 7 insulator. Shaded areas denote boundaries between insulating, metallic and critical MIT regimes. ( d ) Polarized neutron diffraction measurements of Sr 3 Ir 2 O 7 showing radial scans through the Q =(1, 0, 3) superlattice peak at 300 K in both spin-flip (SF) and non-spin-flip (NSF) channels. The magnetic guide field was applied parallel to the momentum transfer Q . Error bars in all plots represent 1 s.d. Full size image The intrinsic crystal structure of Sr 3 Ir 2 O 7 remains an active area of investigation with superlattice reflections violating the tetragonal space group I4/ mmm reported in single-crystal studies [14] , [16] . Previously, our neutron studies resolved high-temperature Bragg scattering [10] at positions forbidden by both the recently reported I4/ mmm (ref. 15 ) and Bbcb (ref. 5 ) space groups. In order to clarify the origin of this high-temperature superlattice, we also performed polarized neutron diffraction measurements with the results plotted in Fig. 3d . Radial scans through Q =(1, 0, 3) show that the (1, 0, L )-type superlattice reflections at 300 K appear only in the non-spin-flip channel with the neutron guide field applied parallel to Q . This demonstrates the structural origin of the superlattice and mandates a space group symmetry lower than Bbcb . The resulting high-temperature (1, 0, L )-type peaks argue for oxygen octahedral tilting as well as in-plane rotation in this system. A tilt already necessarily exists for the c axis-aligned moments in the canted AF phase, and the strong spin-lattice coupling in perovskite iridates [17] supports the notion of an accompanying structural tilt. Such a tilt likely renders Sr-327 isostructural to Ca 3 Ru 2 O 7 (space group: Bb 2 1 m ) [18] ; however, a full neutron data set and structural refinement have yet to be carried out. STS measurements In order to better understand the formation of the metallic phase, low-temperature (4 K) STS measurements were performed on two concentrations: samples with x =0.35 in close proximity to the MIT and samples deep within the metallic regime with x =0.5. 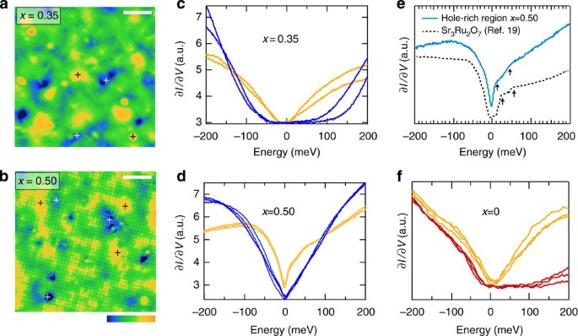Figure 4: STS measurements of Sr3(Ir1−xRux)2O7. (a) Topography at a bias voltage of −100 mV for thex=0.35 concentration near the MIT. (b) Topography at a bias voltage of −100 mV for thex=0.5 metallic concentration. Intensity scales for topography in (a) and (b) are unique to each plot and their relative variation is shown via the colour bar below the panels. White bars in each plot denote the length scale of 3 nm. Colour bar denotes the relative scale of LDOS ranging from low (blue) to high (orange) values. (c) Tunnelling spectra collected in gapped and gapless phase-separated regions denoted by blue and yellow curves collected at white and black crosses in the corresponding map. (d) Spectra forx=0.5 within two regions denoted by yellow and blue curves collected at black and white crosses respectively in the topography. (e) High-resolution tunnelling data collected within a bright region of thex=0.5 sample in (b). Dashed line is low-temperature STS data for Sr3Ru2O7reproduced from ref.19. (f) Spectra collected for Sr3Ir2O7in regions with enhanced LDOS due to oxygen defects (yellow curves) and spectra collected away from defects showing the full charge gap (red curves). We note here that the inhomogeneity observed within the parent insulating system stems from relatively rare regions of oxygen defects and that the majority of the surface showed fully gapped behaviour (red curves), whereas for thex=0.35 andx=0.5 systems the entirety of the samples showed strong electronic inhomogeneity across nanometre-length scales. Figure 4a shows the resulting topography of STS measurements exploring the local density of states (LDOS) in the x =0.35 concentration. Strong inhomogeneity across nanometre-length scales in this sample is immediately apparent from the topography and reveals the coexistence of two distinct local environments whose representative tunnelling spectra are plotted in Fig. 4c . Dark regions with low LDOS in the corresponding map show a fully gapped spectra paralleling that of the parent Sr 3 Ir 2 O 7 insulating phase [7] reproduced in Fig. 4f , while the bright regions reveal metallic regions with an enhanced LDOS. The striking nanoscale coexistence of both fully gapped and gapless metallic regions in this sample demonstrates that the sample segregates into electronically distinct regions. The low-temperature MIT phase line in Fig. 1a therefore does not represent a thermodynamic phase transition but rather the percolation threshold of metallic puddles localized within a spin-orbit Mott phase. Figure 4: STS measurements of Sr 3 (Ir 1− x Ru x ) 2 O 7 . ( a ) Topography at a bias voltage of −100 mV for the x =0.35 concentration near the MIT. ( b ) Topography at a bias voltage of −100 mV for the x =0.5 metallic concentration. Intensity scales for topography in ( a ) and ( b ) are unique to each plot and their relative variation is shown via the colour bar below the panels. White bars in each plot denote the length scale of 3 nm. Colour bar denotes the relative scale of LDOS ranging from low (blue) to high (orange) values. ( c ) Tunnelling spectra collected in gapped and gapless phase-separated regions denoted by blue and yellow curves collected at white and black crosses in the corresponding map. ( d ) Spectra for x =0.5 within two regions denoted by yellow and blue curves collected at black and white crosses respectively in the topography. ( e ) High-resolution tunnelling data collected within a bright region of the x =0.5 sample in ( b ). Dashed line is low-temperature STS data for Sr 3 Ru 2 O 7 reproduced from ref. 19 . ( f ) Spectra collected for Sr 3 Ir 2 O 7 in regions with enhanced LDOS due to oxygen defects (yellow curves) and spectra collected away from defects showing the full charge gap (red curves). We note here that the inhomogeneity observed within the parent insulating system stems from relatively rare regions of oxygen defects and that the majority of the surface showed fully gapped behaviour (red curves), whereas for the x =0.35 and x =0.5 systems the entirety of the samples showed strong electronic inhomogeneity across nanometre-length scales. Full size image In exploring the extent of this segregation between electronic phases or doped carriers further, we performed STS measurements on the metallic x =0.5 concentration. These measurements reveal this sample to be globally gapless; however, the spectra also resolve a substantial degree of electronic inhomogeneity within this nominal metal, as illustrated by a representative topography in Fig. 4b . Correspondingly, the spectra plotted in Fig. 4d again show two distinct shapes representing different local environments: one with suppressed V-shaped LDOS and the second with enhanced LDOS and a spectrum that strongly resembles that of Sr 3 Ru 2 O 7 (ref. 19 ). To better illustrate this, a comparison with Sr 3 Ru 2 O 7 is provided as shown in Fig. 4e . The similarity between the hole-rich regions of the metallic x =0.5 sample and the pure bilayer ruthenate system is particularly striking, with the tunnelling data resembling a thermally broadened version of a qualitatively similar electronic structure. This combined with the strong inhomogeneity of this metallic state indicates that even the fully metallic compounds continue to remain electronically segregated over nanometre-length scales. Our combined experimental results, viewed globally, paint a picture of a nanoscale, electronically phase-separated ground state for in-plane carriers doped within a spin-orbit-driven Mott phase, Sr 3 Ir 2 O 7 ( Fig. 1 ). Since the meaning of ‘electronic phase separation’ is rather subtle at the nanoscale in doped transition metal oxides, we define its use explicitly here simply as the observation of two different local environments with distinct electronic properties. This general scenario of nanoscale phase separation, either via the coexistence of distinct electronic phases or the direct segregation of holes, results in the stabilization of two different local environments and a percolating conduction network sensed by our earlier transport measurements. Bare charge accumulation into puddles of 1–2 nanometre-length scales may not be energetically favourable due to unscreened long-range Coulomb interactions. Without knowing the effective screening length for the Coulomb interaction and the pinning potential for carriers, it is hard to quantify what the length scale should be in Sr 3 Ir 2 O 7 . An alternative of phase separation into electrically neutral, yet electronically distinct, phases separated by a first-order phase transition is instead a likely mechanism; however, we are unable to differentiate this from the pure carrier segregation scenario. Regardless of which scenario dominates, the carriers within metallic patches remain initially localized across ~1–2 nm-length scales, and at the critical concentration where transport measurements show a MIT ( x ~0.35), this leads to the formation of metallic patches percolating within the fully gapped, spin-orbit Mott insulating background. At Ru substitution levels below x =0.35, the thermally driven MIT is therefore the likely result of the expansion of these metallic puddles due to thermal shifts in their free energy relative to insulating host phase. Phase inhomogeneity continues deep into the metallic regime, where our STS data directly demonstrate nanometre-scale texture in metallic Sr 3 IrRuO 7 comprising two distinct regions: (1) large LDOS regions with an electronic response mirroring the 4 d 4 electronic spectrum of isostructural Sr 3 Ru 2 O 7 (ref. 19 ) and (2) regions with V-shaped spectra with LDOS suppressed close to the Fermi energy. Since their valence states are rather far from the Fermi level, A-site doping in perovskite oxides is historically envisioned as controlling the filling of d -bands on the B-sites by donating their valence electrons to the entire system. The resulting doping mechanism gives rise to a rapid suppression of the Mott phase such as in A-site-doped Sr 2 IrO 4 (ref. 20 ) and Sr 3 Ir 2 O 7 (ref. 21 ). Our B-site doping in Sr-327, however, reveals that holes nominally added via Ru substitution remain localized within the IrO 2 planes until ~35% of the Ir 5 d ions have been replaced, close to the classical 2D percolation threshold of 41% (ref. 22 ). Even beyond this threshold at 50% replacement, hole-rich regions remain phase separated. Given that Ru doping is nominally a strong perturbation to the weakly insulating ground state of Sr-327, this observation is striking and suggests that Coulomb interactions and correlation effects remain essential across the majority of the phase diagram of this system. Our combined neutron scattering and STS data reveal that the AF-ordered state that survives across the MIT has a spin–spin correlation length ( ξ >200 Å) that spans across the phase-separated puddles of gapped and metallic regions—revealing a globally AF-ordered phase. Furthermore, in concentrations doped close to the MIT, the recovery of the ordered AF moment to values nearly equalling that of the undoped parent Sr 3 Ir 2 O 7 rules out any trivial superposition of chemically distinct phases. A magnetically ordered, metallic state beyond the MIT is reminiscent of the phase diagrams of (Ca 1− x Sr x ) 3 Ru 2 O 7 (ref. 23 ) and Ca 2− x Sr x RuO 4 (ref. 24 ); however, from our current measurements of Sr 3 (Ir 1− x Ru x ) 2 O 7 the structural symmetry appears identical for concentrations spanning the MIT, suggesting that the critical point is not directly tied to a structural phase transition. AF metallic states have also been proposed in disordered and binary alloy Mott phases as an intermediate state prior to the onset of Anderson localization [25] , [26] . The global picture our data provide shows that the physics here is more complex than that of a trivially diluted AF system with percolative transport. The percolating metallic network seemingly can be induced to order by the host AF matrix, which may explain why the ordered AF moment is actually enhanced near the region of maximum heterogeneous interface area at the MIT as well as why AF order survives across the percolation threshold where no infinite domain of the AF host persists. Local antiferromagnetism does however naively persist across the critical concentration and can continue to influence the metallic phase into the heavily Ru-doped regime. Eventually this gives way to a globally gapless AF phase in the x =0.5 sample. We propose the following picture of magnetic interactions within this system: when they are dilute within the matrix, Ru-doped holes behave in a manner consistent with isolated ions in the S =1 low spin state giving rise to the local moment response; however, increasing the Ru-doping level increases the density of these isolated magnetic impurities, eventually nucleating clusters of metallic regions (resolved directly in our STS measurements). Within these metallic puddles, whose percolation generates the MIT, the local moment should be quenched at low temperatures in a Fermi liquid ground state; however, these puddles may still be magnetically ordered due to proximity of local AF order in neighbouring regions and a large spin susceptibility arising from their nested Fermi surface pockets. Such an instability is indeed known to be present along the Q =(π, π) in-plane wave vectors of Sr 3 Ru 2 O 7 (ref. 27 ) where an enhanced density of states is nested at the Fermi level due to the structural zone folding. In this regard, this suggests similarities to the thermally driven MIT in the prototypical Mott system VO 2 , where percolating metallic puddles display significant correlation effects [28] . More broadly, the survival of an ordered magnetic moment into the metallic state of the system demonstrates that electron–electron correlations remain relevant across the MIT of this system and argues against the picture of Sr 3 Ir 2 O 7 as a trivial band-insulator simply driven by the zone folding that occurs at the onset of AF order. The evolution of AF order across the MIT in the phase diagram of this hole-doped spin-orbit Mott insulator demonstrates that a rich interplay can be realized at the boundary between a novel J eff =1/2 insulator and a correlated metal. The localization of Ru-doped carriers into a phase-separated ground state surprisingly parallels the strongly correlated phase behaviour of 3 d -transition metal oxide systems such as the B-site-doped correlated manganites [29] , [30] , [31] , [32] and reveals that correlation physics can play a dominant role in the electronic phase formation of a doped spin-orbit Mott insulator. Our findings demonstrate that correlation effects felt by carriers introduced within in a 5 d Mott phase remain robust enough to drive electron localization, a key ingredient in emergent phenomena such as high-temperature superconductivity and enhanced ferroic behaviour. This opens up a new frontier for exploring correlated electron phases within the presence of strong SOC effects inherent to a 5 d -electron setting. Materials and crystal growth The single crystals of Sr 3 (Ir 1− x Ru x ) 2 O 7 were grown by conventional flux methods similar to earlier reports [10] , [14] using a SrCl 2 flux. Crystals were grown in platinum crucibles using IrO 2 (99.98%, Alfa Aesar), RuO 2 (99.98%, Alfa Aesar), SrCO 3 (99.99%, Alfa Aesar) and anhydrous SrCl 2 (99.5%, Alfa Aesar) in a 2:3:15 molar ratio. Starting powders were partially sealed inside the crucible with a Pt lid and further contained inside alumina crucibles. Mixtures were heated up to 1,380 °C, cooled to 850 °C at a rate of 3.5 °C per hour, and then furnace-cooled to room temperature. The resulting boule was etched with deionized water and shiny, black Sr 3 (Ir 1− x Ru x ) 2 O 7 crystals with typical dimensions 2 × 2 × 0.1 mm were removed. Ru concentrations were determined to match target values within ~2% via energy-dispersive X-ray spectroscopy (EDS) measurements. EDS measurements were performed on numerous samples across different regions of samples from each growth batch, and measurements were also collected across different length scales to verify chemical homogeneity. Multiple crystals were tested from every batch, and from point to point on a given sample, we were able to resolve a Ru distribution homogenous within a central value ±1% (2% spread). The central value of Ru concentrations between crystals from a single growth batch would vary no more than ±2% from a central value (4% spread). Error bars on the reported phase diagram in the main text reflect this uncertainty—in many cases they are within the symbol size. The actual crystals measured via transport and magnetization measurements and almost all of the crystals for the neutron measurements were first characterized (only the x =0.20 and x =0.15 samples were not, although crystals from the same batch were characterized) via EDS measurements to determine/verify the precise Ru content. X-ray diffraction measurements Single crystals from a single batch of each concentration were ground into a powder and measured via X-ray powder diffraction within a Bruker D2 Phaser diffractometer. X-ray powder diffraction and refinement revealed no impurity phases within instrument resolution (~2–3%). Lattice parameters and unit cell volumes were refined within the I4 /mmm space group and showed both a - and c axes that reduce continuously with increased Ru substitution ( Supplementary Fig. 4 )—as expected, because the smaller Ru 4+ ions are introduced into the lattice. We note here that laboratory-based powder X-ray measurements typically lack the intensity to resolve the known orthorhombic superlattice reflections in this material, so each concentration was instead refined within the tetragonal I4 /mmm space group. Bulk property measurements Magnetotransport measurements were performed via standard four-wire measurements within a Quantum Design PPMS. Magnetization measurements were collected within a Quantum Design SQUID MPMS magnetometer. MIT determined via resistivity The MIT depicted in the phase diagram of Fig. 1a was determined via the temperature at which the slope of the sample’s resistance versus temperature changed sign from to upon cooling. Data showing the MIT for all samples where an MIT was reported are shown in the inset of Fig. 2a and in Supplementary Fig. 1 . Bulk spin susceptibility Local moments were determined via Curie–Weiss fits to the form 1/ χ ( T )=Θ/ C + T / C , where Θ is the Weiss constant and C is the Curie constant (results plotted in Supplementary Fig. 2 ). Here , with N A as Avogadro’s number and k B is Boltzman’s constant. Fits render a negative Weiss constant for x <0.75 consistent with the observation of AF correlations. For x =0.75, low-temperature susceptibility shows the reemergence of an irreversibility temperature ( T irr ) below 20 K. The reentrance of a net ferromagnetic signal in this heavily doped regime is likely the result of the fragility of the nearly magnetic ground state of Sr 3 Ru 2 O 7 where small levels of impurity substitution or pressure are known to stabilize magnetic order [11] . As similar effects are known to occur in Sr 3 Ru 2 O 7 , for the purposes of our study we treat the ground state of x =0.75 as qualitatively similar to that of the ruthenate bilayer end point. We have not performed neutron diffraction measurements exploring the presence of AF order in this concentration. Neutron-scattering measurements The unpolarized neutron diffraction experiments were performed on HB1-A triple-axis spectrometer at the High Flux Isotope Reactor (HFIR) at Oak Ridge National Laboratory (ORNL) and at N-5 triple-axis spectrometer at Canadian Neutron Beam Center, Chalk River Canada. For HB1-A the incident beam was monochromated by the Q =(0, 0, 2) reflection of a double-bounce pyrolitic-graphite (PG) monochromator with a fixed incident energy of E i =14.65 meV, and a PG(002) analyser crystal was used on the scattered side. Two PG filters were placed before the sample, and collimations of 40′–40′–40′–80′ were used before the monochromator, sample, analyser and detector, respectively. Experiments on N5 were performed with a PG monochomator and E i =14.5 meV and PG analyser with one PG filter placed after the sample. Collimations of 30′–60′–33′–144′ were used before the monochromator, sample, analyser and detector, respectively. The polarized neutron experiment was carried out on the BT7 triple-axis spectrometer at the NIST Center for Neutron Research using PG(002) monochromator, 3 He polarizers, PG filters before and after the sample, radial collimation and a position-sensitive detector on the scattered side. A guide field allowed the magnetic field to be tuned along the scattering vector (horizontal field) and perpendicular to the scattering plane (vertical field) configuration. For all experiments, the crystals were aligned in the (H, 0, L) scattering plane. STS measurements Sr 3 (Ir 1− x Ru x ) 2 O 7 single crystals were cleaved at ~77 K in ultra-high vacuum before being directly transferred to the STM head held at 4 K. From previous data, cleaving at low temperatures is critical for obtaining flat clean samples. Tips were prepared by annealing etched W-tips in vacuum and then checking the quality on metallic (copper single crystal) surfaces. The quality of all tips used in this study was checked by imaging standing waves on Cu and performing spectroscopy. The tips thus prepared showed atomic resolution on the iridate samples and were stable, allowing us to obtain high-quality δI/δV maps. Measurement statistics For transport measurements, each batch with a unique Ru concentration was tested at a minimum of three times (in most cases more) on different crystals. Phase transitions determined via transport measurements reproduced within the error bars shown within the phase diagram of Fig. 1a . The most sensitive batches were those with Ru contents close to the sharp MIT phase boundary with x =0.35 where the same slight deviations in Ru content resulted in a larger sample-to-sample variation in T MIT . The resulting uncertainty is encompassed by the horizontal error bars in Fig. 1a , often within the symbol size. For neutron measurements, every data point for T AF on the phase diagram in Fig. 1a represents a measurement on one unique sample. The anomalous regions such as those near the phase boundary with an enhanced moment ( x =0.33–0.35) and deep within the metallic regime ( x =0.5) were checked with additional experiments on additional samples grown in different batches. The magnetic behaviour reproduced in both instances and those data points are not shown. For our magnetization measurements, only a few select samples, well characterized by transport and EDS, were chosen for measurement. Only one measurement was taken for each concentration reported. For STS measurements, for each doping, at least three different tips and samples were studied. The spectral shapes for any given doping were consistent and repeatable. We checked the tip height dependence for the insulating regions of the parent compound and the x =0.35 compound and found no obvious changes in spectral shape with height. We have measured three samples at the x =0.35 concentration and found the reported nanoscale phase coexistence completely reproducible. Three samples with x =0.5 have also been measured and with completely reproducible spectra and surfaces. How to cite this article: Dhital, C. et al . Carrier localization and electronic phase separation in a doped spin-orbit-driven Mott phase in Sr 3 (Ir 1− x Ru x ) 2 O 7 . Nat. Commun. 5:3377 doi: 10.1038/ncomms4377 (2014).